Externally controlled on-demand release of anti-HIV drug using magneto-electric nanoparticles as carriers Although highly active anti-retroviral therapy has resulted in remarkable decline in the morbidity and mortality in AIDS patients, inadequately low delivery of anti-retroviral drugs across the blood–brain barrier results in virus persistence. The capability of high-efficacy-targeted drug delivery and on-demand release remains a formidable task. Here we report an in vitro study to demonstrate the on-demand release of azidothymidine 5′-triphosphate, an anti-human immunodeficiency virus drug, from 30 nm CoFe 2 O 4 @BaTiO 3 magneto-electric nanoparticles by applying a low alternating current magnetic field. Magneto-electric nanoparticles as field-controlled drug carriers offer a unique capability of field-triggered release after crossing the blood–brain barrier. Owing to the intrinsic magnetoelectricity, these nanoparticles can couple external magnetic fields with the electric forces in drug–carrier bonds to enable remotely controlled delivery without exploiting heat. Functional and structural integrity of the drug after the release was confirmed in in vitro experiments with human immunodeficiency virus-infected cells and through atomic force microscopy, spectrophotometry, Fourier transform infrared and mass spectrometry studies. Although highly active anti-retroviral therapy has resulted in remarkable decline in the morbidity and mortality in AIDS patients, zero or inadequately low delivery of anti-retroviral drugs across the blood–brain barrier (BBB) and into the brain and other tissue organs results in virus persistence [1] , [2] , [3] . Hence, the elimination of human immunodeficiency virus-1 (HIV-1) reservoirs still remains a formidable task [4] , [5] . In recent years, use of nanotechnology in medicine has shown exciting prospect for the development of novel remotely controlled drug delivery systems [6] , [7] . Besides magnetic nanoparticles (MNs) [8] , [9] , [10] , other delivery systems rely on using thermally responsive polymers, optically (ultraviolet (UV), visible wavelength and IR) and acoustically activated nanostructures, liposomes, electrochemical processes and others. An extensive review of these and other active triggering approaches was presented in the article by Timko et al. [11] . The unique advantages of magnetically forced triggering place this approach in a class of its own. In this case, the speed of delivery is determined by the external magnetic field. For instance, as it is related to the delivery across the BBB, this approach provides a way to deliver drugs sufficiently fast to avoid their engulfing by the reticuloendothelial system. Nucleotide reverse transcriptase inhibitor 3′-azido-3′-deoxythymidine-5′-triphosphate (AZTTP) is among the most challenging anti-retroviral drugs to deliver across the BBB [12] , [13] . Previously we have shown that MNs tagged with AZTTP transmigrated across the BBB by the application of an external magnetic field without affecting the integrity of the BBB, and the transmigrated AZTTP demonstrated significant inhibition of HIV-1 p24 antigen production in an in vitro infection model system compared with the free AZTTP [14] . However, this MN-based delivery suffers from the lack of certainty of drug release from the carrier if and when the nano-carrier reaches the target. The current presumptive mechanisms of drug delivery depend on manually uncontrollable cellular phenomena such as exocytosis of drug containing intracellular vesicle, intracellular Ca 2+ concentrations and pathology-specific responses (change in pH, temperature, and so on) [15] . As a result, to obtain a relatively small physiologic change and to ensure the release of the drug, the binding force between the nano-carrier and the drug must be maintained relatively weak. Consequently, more than 99% of the drug/carriers are deposited in the liver, lungs and other lymphoid organs before they reach the target. Therefore, an approach for finely controlled and enhanced release of AZTTP in sufficient therapeutic levels in the brain or in other target organs is still sought after, as it is critical for the complete eradication of HIV. We present a study to demonstrate that dissipation-free, energy-efficient and low-field on-demand drug release can be achieved if the conventional MN carriers are replaced by magneto-electric (ME) nanoparticles (MENs) [16] . ME materials represent a relatively recently introduced class of multi-functional nanostructures in which magnetic and electric fields can be strongly coupled at body temperature [17] . Similar to the MNs, MENs can be designed to have adequately high magnetic moments and, therefore, also can be used for targeted delivery by applying remote direct current (d.c.) magnetic fields. However, owing to their non-zero magneto-electricity, unlike the traditional MNs, MENs offer an additional feature that can enable a new dissipation-free mechanism to force a high-efficacy externally controlled drug release process at the sub-cellular level using remote low-energy d.c. and/or alternating current (a.c.) magnetic fields. An exaggerated illustration in Fig. 1 explains the concept of the field-triggered on-demand drug release from MENs. To simplify the description, we use an example with a remote magnetic field in one specific direction, for example, along x axis, with respect to the MEN drug nano-complex. The original (zero field) ionic bond, with charge Q ionic of the nanoparticle, is schematically shown in Fig. 1a . AZTTP molecules (typically interconnected in chains) surround each MEN in a symmetric manner. As shown in Fig. 1b , as a non-zero magnetic field is applied, a non-zero electric dipole moment is formed in the nanoparticle because of the non-zero ME effect. For simplicity assuming an isotropic model, the triggered dipole moment Δ P=αH , where α is the first order ME coefficient and H is the magnetic field. The amplitude of the dipole charge surface density on each side of the nanoparticle along the field would be of the order of σ ME ~± αH, where ‘positive’ and ‘negative’ signs are applied to the opposite sides of the dipole, respectively. The dipole moment breaks the original symmetry of the charge in the MEN shell. Consequently, as the magnitude of the magnetic field is further increased above the threshold value at which the dipole charge density on the ‘negative’ side becomes comparable to the positive ionic charge density in the shell, σ ME ~ Q ionic / πd 2 , that is, H th ~Q ionic /πd 2 α , where d is the diameter of the MEN, the bond in this direction along the x axis will be broken while the opposite bond will be further strengthened, as illustrated in Fig. 1c . By symmetry, to break the bond in the opposite direction, the field sequence should be repeated in the reverse direction, as illustrated in Fig. 1d . This simplified scenario doesn’t take into account the randomness of the orientations of the nanoformulations. Ideally, applying an a.c. magnetic field that equivalently sweeps all bond orientations will create a more uniform and efficient bond-breaking process over the surface of the nanoformulation, and thus enhance the drug release efficacy. In the next generation of the technology, this goal can be achieved by using a spatially rotating field, which in turn can be accomplished, for example, by using an array of coils that generate a.c. fields with non-zero phase shifts with respect to each other. 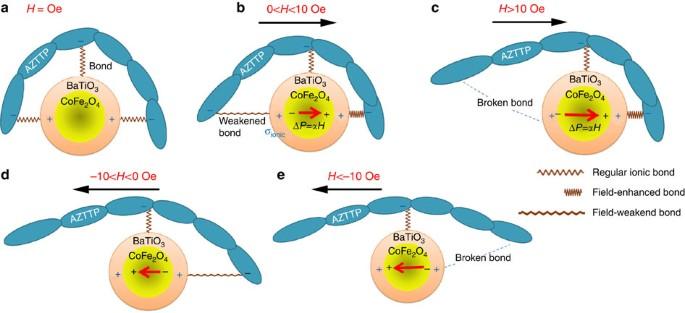Figure 1: Illustration of the underlying physics of the a.c.-field-triggered release. A simplified (one directional) illustration of the concept of on-demand drug (AZTTP) release by MENs stimulated by a uniform a.c. magnetic field in X direction. (a) At zero field, only the ionic charge is present in the MEN shell. (b) An additional dipole moment (proportional to the magnetic field) breaks the original symmetry of the charge distribution in the shell. (c) As the field is increased above the threshold value (σionic~σME), the bond on one side is broken. (d,e) The field is reversed to break the bond on the opposite side of the nanoparticle. The red arrows show the electric dipole due to the ME effect. In practice, owing to the random configurations of nanoformulations with respect to the field, the effect is present along every central bond orientation. Figure 1: Illustration of the underlying physics of the a.c.-field-triggered release. A simplified (one directional) illustration of the concept of on-demand drug (AZTTP) release by MENs stimulated by a uniform a.c. magnetic field in X direction. ( a ) At zero field, only the ionic charge is present in the MEN shell. ( b ) An additional dipole moment (proportional to the magnetic field) breaks the original symmetry of the charge distribution in the shell. ( c ) As the field is increased above the threshold value ( σ ionic ~ σ ME ), the bond on one side is broken. ( d , e ) The field is reversed to break the bond on the opposite side of the nanoparticle. The red arrows show the electric dipole due to the ME effect. In practice, owing to the random configurations of nanoformulations with respect to the field, the effect is present along every central bond orientation. Full size image In this study, we verified the hypothesis by demonstrating the on-demand release of AZTTP from 30-nm CoFe 2 O 4 @BaTiO 3 MENs by applying low a.c. and d.c. magnetic fields. We showed that a 44 Oe a.c. field at 1,000 Hz was sufficient to trigger over 89% release. Further, to support the dissipation-free release model, we could use a 66 Oe d.c. field to trigger a comparable release level. Design of the experiment We used atomic force microscopy (AFM) in conjunction with UV spectrophotometry, Fourier transform infrared (FTIR) analysis and mass spectroscopy to directly trace the kinetics of the drug release process at different stages of the release under the influence of remote d.c. and a.c. magnetic fields. The three key stages included (i) the initial state with separate MEN carriers and AZTTP molecules, (ii) the loaded state in which MEN drug nanoformulations are formed and (iii) the final state after the a.c.-field-forced separation of AZTTP and MENs, that is, after the on-demand drug release. In vitro experiments on HIV-infected human cells were conducted to demonstrate the structural and functional integrity of AZTTP after this physical release process. Below we present the key results of this experimental study. The experiments are described in more detail in the methods section. Transmission electron microscopy study of MENs In the experiments described below, for the role of MENs we used nanoparticles made of the popular core–shell composition CoFe 2 O 4 @BaTiO 3 , in which the relatively high moment CoFe 2 O 4 1-nm shell was used to enhance the ME coefficient [18] . In general, nanoparticles as small as 5 nm in diameter can be fabricated with physical methods such as ion beam proximity lithography or imprint lithography [19] . In this study, considering the novelty of the approach, we focused on the main discovery of using MENs for on-demand drug release rather than on the development of scaling approaches. The default measurements were conducted with 30-nm MENs. A typical transmission electron microscopy image of the fabricated MENs, with clearly visible core–shell structures, is shown in Fig. 2a . The composition of the MENs was confirmed through energy-dispersive spectroscopy, as shown in Fig. 2b . The ME coefficient for the nanoparticles was measured via point I–V methods in the presence of a field to be the order of 100 V cm −1 Oe −1 , using an approach described in our previous publication [20] . 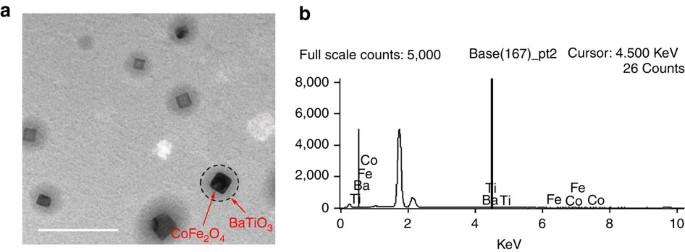Figure 2: Transmission electron microscopy (TEM) analysis of MENs. (a) A TEM image of MENs. The core–shell structure of a MEN is highlighted. Scale bar, 100 nm. (b) An energy-dispersive spectroscopy (EDS) analysis of MENs. Figure 2: Transmission electron microscopy (TEM) analysis of MENs. ( a ) A TEM image of MENs. The core–shell structure of a MEN is highlighted. Scale bar, 100 nm. ( b ) An energy-dispersive spectroscopy (EDS) analysis of MENs. Full size image Spectrophotometry study of the release The goal of the first experiment was to measure the amount of the drug (AZTTP) at different stages of the release process using the conventional approach of spectrophotometry by measuring the UV light absorption at the 267 nm maximum of the drug’s absorption spectrum. We could bind ~24% of the drug to the nanoparticles by incubating AZTTP with the MENs in the Tris-EDTA (TE) buffer (pH 7.4) for 3 h. The amount of the bound drug was determined by estimating the concentration of AZTTP in the unbound fraction (supernatant) of the incubation mixture by spectrophotometry. To apply remote d.c. and a.c. magnetic fields, we used a low-energy low-field Helmholtz pair connected to a function generator. The chart in Fig. 3 summarizes the key results of this experiment, in which we measured the amount of the unbound drug depending on the external field strength and frequency. It can be seen that application of a 44 Oe field at 1,000 Hz results in 89.3% of the drug being released, while application of a d.c. field of the same amplitude releases only 16.4% of the drug. The data also confirm that with higher frequency, a lower magnetic field is needed to break the bonds because oscillation of the bonds caused by a higher frequency field facilitates the breaking of the bonds. However, when a strong enough d.c. field (>~65 Oe) is applied, the bond-breaking side of the drug chain can gain enough momentum, causing the chain to break free from the MEN shell even at zero frequency. To fully exploit the potential of the new controlled drug release nanotechnology, it is important to conduct a more detailed pharmacokinetics study. 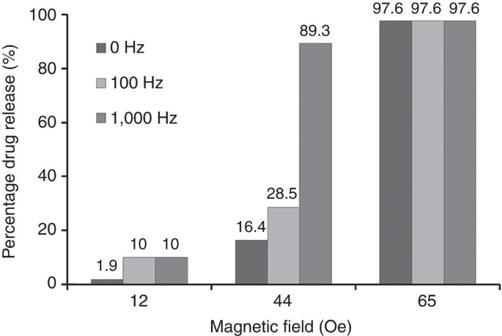Figure 3: Field strength and frequency dependence of the drug release. Chart showing the release efficacy of AZTTP drug bound to MENs by a remote magnetic field at different amplitudes and frequencies. Figure 3: Field strength and frequency dependence of the drug release. Chart showing the release efficacy of AZTTP drug bound to MENs by a remote magnetic field at different amplitudes and frequencies. Full size image Pharmacokinetics study In this experiment, MENs loaded with AZTTP drug were exposed to an external magnetic field at different strengths (12, 44 and 66 Oe) and frequencies (0, 100, 1,000 Hz) for different treatment durations (1, 5, 10, 60 and 120 min) in order to understand the release kinetics. Results are summarized in the three-dimensional chart in Fig. 4 . The quantitative values are also presented in Supplementary Table S1 . For every field–frequency combination set we used a fresh solution with AZTTP-loaded MENs. 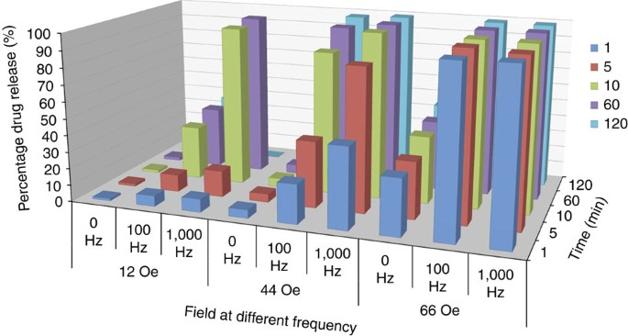Figure 4: Pharmacokinetics study. Pharmacokinetics study: three-dimensional chart representation of the drug release percentage at various combinations of the field strength (12, 44 and 66 Oe), the frequency (0, 100, and 1,000 Hz) and the treatment duration (1, 5, 10, 60 and 120 min). Figure 4: Pharmacokinetics study. Pharmacokinetics study: three-dimensional chart representation of the drug release percentage at various combinations of the field strength (12, 44 and 66 Oe), the frequency (0, 100, and 1,000 Hz) and the treatment duration (1, 5, 10, 60 and 120 min). Full size image FTIR analysis The concept of the drug release by a remote magnetic field was confirmed also through FTIR analysis, as shown for the three key stages of the process kinetics in Fig. 5 : (top) free MENs and AZTTP before loading, (middle) loaded state: MEN–AZTTP nanoformulations and (bottom) MENs after the AZTTP release by a remote 44 Oe field at a 100 Hz frequency. Compared with the initial and final unbound states, the loaded state showed almost 30% weaker absorbance in general and a transformed spectrum in the wavenumber region from 1,750 to 1,250 cm −1 . 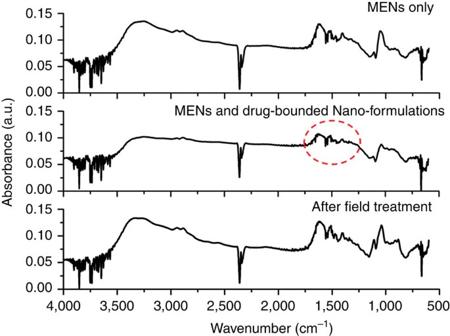Figure 5: FTIR measurements. FTIR measurements for MEN–AZTTP system at three different stages: (i) (top) MENs only, (ii) (middle) AZTTP-loaded MENs and (iii) MENs after the release by the a.c. field treatment (bottom). Figure 5: FTIR measurements. FTIR measurements for MEN–AZTTP system at three different stages: (i) (top) MENs only, (ii) (middle) AZTTP-loaded MENs and (iii) MENs after the release by the a.c. field treatment (bottom). Full size image AFM study of the release kinetics To observe the release process at the molecular level, we conducted the following AFM measurements. 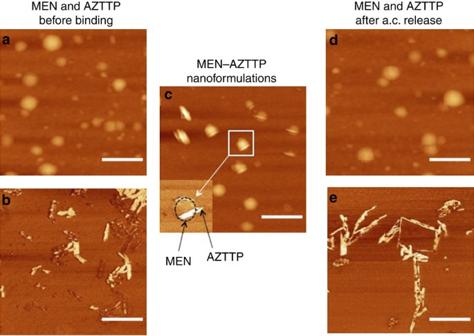Figure 6: Atomic force microscopy study of the drug release kinetics. AFM images at different stages of the release process: (a) MENs and (b) AZTTP chains before the loading (binding) step, (c) AZTTP–MEN nanoformulations after the loading process, (d) MENs and (e) AZTTP after the drug release by a 44-Oe a.c. field at 1,000 Hz. Scale bar, 100 nm. Figure 6 shows a sequence of AFM images that reflect the following four stages of the release process: free (a) MEN and (b) AZTTP chains, (c) loaded MEN–AZTTP nanoformulations, and (d) MENs and (e) AZTTP after the release by a 44-Oe a.c. field at 1,000 Hz. To obtain images c and d, the unloaded drug was washed away with the supernatant. One can observe that the MENs and AZTTP chains before the loading step and after the release process look similar. Figure 6: Atomic force microscopy study of the drug release kinetics. AFM images at different stages of the release process: ( a ) MENs and ( b ) AZTTP chains before the loading (binding) step, ( c ) AZTTP–MEN nanoformulations after the loading process, ( d ) MENs and ( e ) AZTTP after the drug release by a 44-Oe a.c. field at 1,000 Hz. Scale bar, 100 nm. Full size image Field-controlled delivery and drug release by MENs Translocation experiments were performed on day 5 of BBB cell culture. In order to achieve the translocation of AZTTP across the BBB, AZTTP were loaded on MENs and subjected to an external magnetic field of 40 Oe (to avoid any unwanted drug release at higher fields) for 3 h and a gradient of ~22 Oe cm −1 (to pull the nanoparticles across the BBB) for 6 h of the incubation period. To apply a field normal to the BBB, the field coils were placed below the cell culture wells carrying the BBB model. Once the incubation was completed, the medium in the bottom chamber was isolated and subjected to the a.c. magnetic field (66 Oe at 100 Hz field for 5 min) to increase the release percentage. After the field treatment, the MENs were isolated via a magnetic separation technique. Once separated, the supernatant was measured for the drug concentration via spectrophotometry. The results indicated that ~40% of the drug was translocated across the BBB as a result of the process. These results are summarized in Supplementary Fig. S1 . To further confirm the structural and functional integrity of the drug after the a.c. release process, we conducted: (i) a mass spectrometry analysis of the drug before and after the release ( Supplementary Fig. S2 and Supplementary Table S2 ), (ii) an in vitro experiment to study the p24 inhibition efficacy of the drug before and after the release ( Supplementary Fig. S3 ). Finally, to understand the cytotoxicity of MENs (CoFe 2 O 4 @BaTiO 3 ), we performed an XTT (sodium 2,3,-bis(2-methoxy-4-nitro-5-sulfophenyl)-5-[(phenylamino)-carbonyl]-2H-tetrazolium inner salt) assay on human astrocyte (HA) cells for neural cytotoxicity and on human peripheral blood mononuclear cells (PBMCs) for peripheral cytotoxicity. The results indicated no significant toxicity at a concentration of <50 μg ml −1 ( Supplementary Table S3 ). The spectrophotometry experiment ( Fig. 3 ) indicates the threshold value, necessary for the field to start the release of the AZTTP drugs by the MENs, to be of the order of 10 Oe, even though only 10% of the drug was released at such a low field value. Using the simplified expression we derived above for the release threshold field ( H th ~Q ionic /πd 2 α ) and assuming the nanoparticle diameter ( d =30 nm) and the ME coefficient ( α =100 V cm −1 Oe −1 ), we can evaluate the value for the effective charge, Q ionic (responsible for the ionic/covalent bond between the MEN and AZTTP cluster), to be ~10 −17 C. The estimate seems reasonable and indicates that approximately a few hundred electrons are involved in the bond formation. Further, in agreement with the original hypothesis, the experiment also proves that the a.c. field provides a substantially more enhanced release compared with that of the d.c. field. Indeed, at 12 Oe field amplitude, d.c. and a.c. (100 Hz) fields result in 1.9 and 10% released drug percentage, respectively. To achieve almost full (89.3%) drug release, a field of 44 Oe at a frequency of 1,000 Hz is required. The effect of the a.c. field control is significant in this case. For comparison, with a field of 44 Oe at the frequency of 100 Hz, the released amount was 28.5% while for the d.c. case at the same field amplitude was only 16.4%. The experiment indicates that such nanoformulations can be directed to the targeted cells via a d.c. magnetic field with a spatial gradient while the drug can be effectively released on demand via an external a.c. magnetic field at 1,000 Hz. Note that the highest applied field of 65 Oe immediately saturated the system, resulting in an almost full drug release even in the d.c. case. According to our hypothesis, the latter can be explained by the magnetic-field-triggered large electric force that gave enough momentum to break the bond. The results of the more detailed pharmacokinetics study ( Fig. 4 ) also indicate the presence of a certain threshold field that needs to be applied to trigger the release. The threshold values at different frequencies reach their saturation value in about 60 min of the incubation process. Again, this threshold field exists even in the d.c. case (zero frequency) and can be further reduced in the a.c. case by increasing the frequency of an a.c. field. To separate the d.c. and a.c. functions for drug delivery and release, respectively, it is important to maintain the amplitude of the field below the saturation value, for example, at 44 Oe. This separation of the d.c.- and a.c.-driven delivery and release functions, respectively, was also confirmed in the in vitro experiment with a human BBB cell culture ( Supplementary Fig. S2 ). The FTIR results are in agreement with spectrophotometry data ( Fig. 5 ). Supporting the above release model, the initial state (before drug loading) and the final state (after the release) FTIR spectra look similar, while the altered intermediate state reflects the effect of binding between MENs and AZTTP molecules. The AFM measurements ( Fig. 6 ) directly illustrate the physical difference between MEN–AZTTP nanoformulations and the free MENs before loading and after releasing the drugs. In agreement with the described spectrophotometry and FTIR measurements, the AFM analysis also indicates that the MENs return to their original unbound state after the drug release triggered by a.c. magnetic field. In addition, AFM also proves the nanoscale nature of the approach, with the potential to be applied at the sub-cellular level. The in vitro experiment using human PBMCs infected with HIV-1 Ba-L proves the intact integrity of the drug after the a.c.-triggered release ( Supplementary Fig. S3 ). The fundamental difference between MNs and MENs is due to the presence in the latter of the quantum-mechanically caused ME effect that enables intrinsic coupling between the magnetic spin and the electric dipole. Consequently, energy-efficient and dissipation-free remote control of the intrinsic charge distribution in the MENs (and consequently, control of the bonding force between the MENs and the drug) can be enabled via application of an external magnetic field. Because of the intrinsic ME effect, even if the drug is strongly bonded to the MEN carriers (as required for high-efficacy delivery), it can be fully released at the target location via application of a local magnetic field with a strength above a certain threshold defined by the ME effect. For comparison, the drug release process using the conventional MNs is not controlled at the same fundamental level but instead is based on an irreversible energy dissipation process caused by an external a.c. magnetic field. In one MN implementation, superparamagnetic nanoparticles and drug molecules are incorporated into temperature-sensitive synthetic polymers or other biomaterials that release the drug as the nanoparticles are heated under the field exposure [21] . In other implementations, superparamagnetic nanoparticles can be coated with intermediate linkers (tailored to specific load molecules), embedded in a ferro-gel, or directly connected to the load molecules [22] , [23] . In either of these conventional cases, the release mechanism with MNs is based on extrinsic phenomena, that is, mechanical deformation and/or heat dissipation that affects the release kinetics, that are triggered by a relatively high frequency a.c. field (in the range of hundreds of kilohertz or above) and consume a substantial amount of power (in the kilowatt range). On the contrary, the MEN-triggered release process is achieved at the intrinsic level and does not require any intermediate materials. It is dissipation free and extremely energy efficient. The release with MENs can be triggered by an a.c. magnetic field at a relatively low frequency (below 100 Hz) and even at a d.c. field provided the field strength is above a certain threshold value, as described below in more detail, with power consumption in the sub-watt range. One can argue that MENs may also experience the potential problem of having a relatively large fraction of the nanoparticles (together or without the drug) trapped in the reticuloendothelial system. One solution to this problem is to apply a ‘zig–zag’-shaped time-varying field profile to move the nanoparticles through the system. Then, besides the force along the main delivery path, there is a significant ‘jolting’ force normal to this direction. This ‘jolting’ force ensures that the nanoparticles don’t become trapped in the fibres of the reticular connective tissue. However, application of the strongly inertial ‘zig–zag’ force to the conventional MNs can also result in a significant loss of the drug. On the contrary, with MENs, the physical bond between the drug and the nanoparticle can be engineered to be adequately strong to avoid any loss until a command to release is given via an external field. As a final remark, we would like to emphasize that although MENs indeed have a unique advantage of serving in both roles, (i) as regular MNs for drug delivery (via application of a d.c. remote field with a spatial gradient) and (ii) as drug release nanoscale sites, their capability of an on-demand drug release by application of a low remote magnetic field in an extremely low frequency range is unprecedented and therefore is a merit of its own (even without exploiting the drug delivery feature). In general, this physically controlled release method could be complementary to any other drug delivery and tagging mechanism, whether it is physical or chemical. Although AZTTP is used in the experiment, the ability of on-demand drug release by a MEN nano-carrier discovered in this study is also relevant to the treatment of other diseases such as many CNS diseases, cancer and others, where deep-tissue high-efficacy drug delivery at the sub-cellular level is key [12] . Preparation of CoFe2O4-BaTiO3 core–shell MENs CoFe 2 O 4 nanoparticles were prepared by hydrothermal method. In this method, 15 ml of aqueous mixture of 0.058 g of Co(NO 3 ) 2 .6H 2 0, 0.16 g of Fe(NO 3 ) 3 .9H 2 0 and 0.2 g of polyvinylpyrrolidone is dissolved in 5 ml of aqueous 0.9 g of sodium borohydride at 120 °C for 12 h. Next, precursor solution of BaTiO 3 was prepared by mixing 30 ml of aqueous 0.029 g of BaCO 3 and 0.1 g of citric acid with 30 ml of ethonalic solution of 0.048 ml titanium isopropoxide and 1 g of citric acid. CoFe 2 O 4 @BaTiO 3 core–shell MENs are prepared by dispersing 0.1 g of CoFe 2 O 4 nanoparticles in the precursor solution. The mixture was sonicated for 2 h. Well-dispersed mixture was dried at 60 °C for overnight while stirring continuously. Later, the mixture was subjected to calcination at 780 °C for 5 h. By reducing the cooling rate (controlled by furnace CMF 1,100) from above 52 to below 14 °C min −1 , the average diameter of MENs could be controlled from below 25 nm to over 100 nm, respectively, with an adequate size distribution of <30%. The particle size distribution was measured by a Zetasizer Nano series via the standard dynamic light scattering approach. For the 25-nm process (14 °C min −1 cooling rate), the average size distribution ranged from ~19 to 31 nm. Nanoformulations of AZTTP–MEN Ten microlitres of AZTTP drug (10 mM, concentration) was added to the solution of 190 μl of TE buffer and 50 μl of CoFe 2 O 4 BaTiO 3 core–shell MENs (5 mg ml −1 ). Then, the solutions were incubated for 2and 3 h, respectively. After the incubation, the solution was subjected to the magnetic field in order to precipitate the MENs (conjugated with AZTTP). After the supernatant was isolated, its absorption was measured at 267 nm using spectrophotometer Agilent Cary 100. Spectro-photometric analysis of drug loading Drug loading percentage=(absorbance of total amount of drug used—absorbance of drug used in supernatant after incubating the drug and the MEN for a specific incubation time) × 100%. After 2-h incubation, the percentage of the drug in the supernatant was ~89%, which corresponded to ~11% (100−89) of the drug bound to the MENs. After 3-h incubation, the percentage of the drug in the supernatant was ~76%, which corresponded to ~24% (100−76) of the drug bound to the MENs. Drug release percentage: drug release percentage=(absorbance of supernatant after magnetic field treatment)/(absorbance of supernatant after incubating the particles with drug) × 100%. The absorbance signal was measured at the maximum wavelength of 267 nm. Magnetic field treatment To eliminate any potential residual unbounded drug, after isolating the supernatant, the precipitate of the MENs conjugated with the drug was washed once with the TE buffer. Then, the drug-conjugated particles (AZTTP–MEN nanoformulations) were redispersed in 190 μl of the TE buffer, and subjected to a magnetic field of varying field strength and frequency. Finally, the solution was precipitated to pipette out the supernatant for further absorption measurements. Surface charge of MENs and AZTTP molecules Because of the triphosphate functional groups, in the chemical (covalent and/or ionic) bond between the MENs and the AZTTP molecular cluster chains, the CoFe 2 O 4 -BaTiO 3 MENs and the AZTTP chains were positively and negatively charged, respectively. Mass spectrometry analysis of AZTTP molecules and AZTTP bound to MEN To confirm the integrity of AZTTP (C 10 H 16 N 5 O 13 P 3 ; MW=507) drug after the a.c.-triggered release by MENs, we conducted a mass spectrometry analysis. The analysis included a full scan qualitative identification of the target analyte, a chromatographic separation and an assessment of the presence of the drug in the composite material (AZTTP–MEN nanoformulations) using multiple reaction monitoring for appropriate transitions. Different mixes were contained in Eppendorf vials. Using a 100-μl micropipette, 100 μl of each vial was transferred to a new disposable polypropylene 96-well plate (part no. 5042-1386). The vials’ contents were subjected to a flow injection analysis using electrospray ionization with Jet Stream Technology in both positive and negative mode to assess the presence of the AZTTP drug. The measurements were conducted with mass spectrometer Agilent LC/MS Triple quadruple G6460 LC-QQQ. The ionization conditions are presented in Supplementary Table S2 . Supplementary Figure 2 shows the number of counts versus the mass-to-charge ratio for the three key stages of the release process: (top) standard AZTTP, (middle) AZTTP bound to MENs, and (bottom) AZTTP and MEN after the a.c.-triggered release of the drug load. The molecular weight of the AZTTP molecule is ~507. Preparation of samples for AFM and FTIR imaging Ten microlitres of AZTTP drug (10 mM, concentration) was added to the solution of 190 μl of the TE buffer and 50 μl of CoFe 2 O 4 -BaTiO 3 core–shell MENs (5 mg ml −1 ). Then, the solution was incubated for 3 h. After the incubation, one drop of solution was air dried on to a pre-cleaned Si wafer. Once dried AFM imaging (topography and phase contrast) was performed using Nanoscope IIIa Multimode. For AZTTP the above solution without MENs was used and for MENs the above solution without AZTTP was used. For FTIR measurements, the sample preparation procedures were similar to the one used for AFM. In vitro BBB model In vitro BBB model was prepared according to the procedure described elsewhere [24] . The BBB model consisted of two compartments (upper and lower), which were separated by the polyethylene terephthalate membrane of a 3.0-μm pore size (Becton Dickinson Labware, NJ, USA). In a 24-well cell culture inserts, 2 × 10 5 human brain microvascular endothelial cells were grown to confluence on the upper side of the insert and the same amount of HAs were grown on the underside. BBB cell culture was incubated for 4 days in order to reach incubation confluence at 37 °C and 5% CO 2 . Transendothelial electrical resistance was used to measure the intactness of the BBB. The average transendothelial electrical resistance value for individual BBB was about 150–200 ohms cm −2 , which is consistent with formation of BBB. p24 Assay to confirm the integrity of AZTTP after field-controlled release Normal PBMCs (10 × 10 6 cells) were infected with native HIV-1 Ba-L (NIH AIDS Research and Reference Reagent Programme catalogue no. 510) at a concentration of 2 ng ml −1 cells for 2 h, washed with phosphate-buffered saline (GIBCO-BRL, Grand Island, NY) and returned to culture with and without fresh (new) or MEN-released AZTTP at equimolar concentrations (200 nM). The culture supernatants were quantitated for p24 antigen using a p24 ELISA kit (ZeptoMetrix, Buffalo, NY) on the 5th day of infection. While the control sample showed the p24 concentration of ~33,050 pg ml −1 , the use of fresh and MEN-released AZTTP drugs resulted in the concentration values of ~1,300 and 1,800 pg ml −1 , respectively ( Supplementary Fig. S3 ). Therefore, considering the s.d. of ~300 pg ml −1 , the two drug forms demonstrated equal p24 inhibition efficacy. In vitro cytotoxicity assay To understand the in vitro cytotoxicity of MENs (CoFe 2 O 4 @BaTiO 3 ), we performed XTT assay according to the manufacturer’s protocol (ATCC). XTT is a quantitative colorimetric assay, which is based on the formation of an orange-coloured formazan dye by viable cells from the cleavage of XTT tetrazolium salts. The assay was performed on HA cells for neuronal cytotoxicity and on PBMCs for peripheral cytotoxicity. In this assay, desired cells were seeded in a 96-well cell culture plate at a 1 × 10 5 cells per well concentration and incubated for 48 h. (The cell concentration and incubation time were standardized by performing a pre-assay optimization protocol.) Following the incubation, the cell culture medium was replaced by a medium containing MENs at a differential concentration of 0–50 μg ml −1 . The cells were incubated in the MEN solution for 24 h. Once, the incubation period was completed the cells were washed with phosphate-buffered saline buffer and later supplemented with a fresh medium. Cell viability test was performed by XTT test kit as supplied by (ATCC) for 6 h. The experiments that were performed in triplicate indicated no significant toxicity at a concentration of <50 μg ml −1 ( Supplementary Table S3 ). How to cite this article: Guduru, R. et al. Externally controlled on-demand release of anti-HIV drug using magneto-electric nanoparticles as carriers. Nat. Commun. 4:1707 doi: 10.1038/ncomms2717 (2013).